Circadian rhythm reprogramming during lung inflammation Circadian rhythms are known to regulate immune responses in healthy animals, but it is unclear whether they persist during acute illnesses where clock gene expression is disrupted by systemic inflammation. Here we use a genome-wide approach to investigate circadian gene and metabolite expression in the lungs of endotoxemic mice and find that novel cellular and molecular circadian rhythms are elicited in this setting. The endotoxin-specific circadian programme exhibits unique features, including a divergent group of rhythmic genes and metabolites compared with the basal state and a distinct periodicity and phase distribution. At the cellular level, endotoxin treatment also alters circadian rhythms of leukocyte counts within the lung in a bmal1 -dependent manner, such that granulocytes rather than lymphocytes become the dominant oscillating cell type. Our results show that inflammation produces a complex re-organization of cellular and molecular circadian rhythms that are relevant to early events in lung injury. Circadian rhythms are daily fluctuations in biological activity that help organisms adapt to their environment [1] . They can be observed at all levels of biology, from behaviour to the abundance of biomolecules, and have a strong genetic basis. One of the major advances in recent years in understanding how circadian rhythms form was the elucidation of the ‘molecular clock’, a transcriptional network that is critical for circadian rhythm generation in healthy mammals [2] , [3] . At the organism level, the molecular clock is organized in a hierarchy, composed of ‘master clocks’ in the hypothalamus that synchronize the oscillations of local clocks residing in peripheral organs [4] . Peripheral circadian clocks influence gene expression in a tissue-specific manner and are responsible for tailoring circadian regulation to the physiologic function of different organs [5] , [6] . With the acceptance of the molecular clock as a paradigm, it has become common practice to use the rhythmic expression patterns of clock genes as surrogate markers for circadian rhythms in general. This has led to the theory that circadian regulation is disabled during acute inflammatory states, because challenging rodents or human subjects with endotoxin or bacteria leads to widespread disruptions in clock gene expression [7] , [8] , [9] . Although it is known that circadian rhythms regulate the inflammatory response of healthy organisms when they initially encounter a pathogen [9] , current theory assumes that circadian rhythms are lost at the molecular level once systemic inflammation ensues. We were interested in this assumption because the molecular clock paradigm was developed by studying organisms in the basal state only. There is little direct evidence that the regulatory networks needed to achieve circadian rhythms in the basal state are equally critical during inflammation. Therefore, disruptions to clock gene expression during inflammation might not necessarily equate with global disruption of circadian rhythms as theorized. The major obstacle is that there are currently no data sets to establish whether or not circadian regulatory patterns occur during systemic inflammation, prompting some authors to call for genome-wide analyses [10] . To this end, we used a genome-wide approach to analyse circadian patterns of regulation in the lungs of mice subjected to endotoxemia. We chose the lung because it represents a primary portal for systemic infection and organ failure in critically ill patients, and because the lung exhibits strong physiological circadian rhythms in health and in diseases such as asthma [11] , [12] . We found that endotoxemic lungs harbour an intricate system of circadian regulation that reprogrammes temporal relationships between gene expression, metabolites and leukocyte trafficking within the inflamed lung. A data set to examine lung circadian rhythms in mice To examine circadian rhythms in mouse lung, we generated a core data set consisting of two independent time-series experiments ( Supplementary Fig. 1a ). This approach enabled us to identify circadian gene expression that was both reproducible and independent of food and light cues. Lungs from one of the time series (Experiment 2) were further used for metabolite measurements and immunohistochemistry (IHC; see Methods), enabling correlations between circadian gene expression, metabolites and lung architecture. In addition, a subgroup of mice from this experiment was subjected to endotoxemia ( Supplementary Fig. 1a ). We were interested in three kinds of gene expression patterns: oscillatory expression that occurred exclusively under basal conditions, gene expression that retained circadian variation regardless of health state and, if present, gene expression that developed oscillatory expression only during endotoxemia. We followed the standard convention of reporting times of day in units of circadian time (CT), where CT0 represents lights-on and CT12 lights-off. 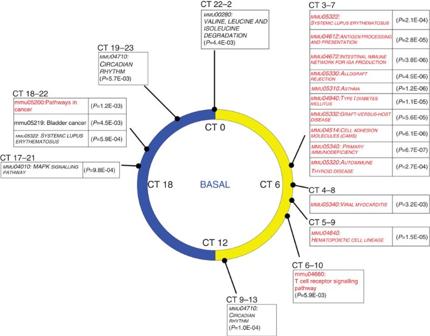Figure 1: Temporal map of KEGG terms enriched in the basal circadian transcriptome of mouse lung. The 4-h phase interval that returned the lowest enrichmentP-value (EASE score modification of the Fisher exact test61) for a given KEGG term was used to position that term on the map. Time of day is expressed in ‘CT’, with CT0 representing the beginning of the light phase and CT12 the beginning of the dark phase. Terms that were also enriched in the master list of 1,190 probes (without consideration of acrophase) are bolded and in caps. Terms whose enrichment atP<0.05 depended on the inclusion of leukocyte-associated genes (see Methods) are coloured red. For clarity, only terms with enrichmentP-values <0.01 are depicted. Note for two KEGG Terms (Circadian Rhythm and Systemic Lupus Erythemasosis), there were two optima inP-values in the basal state and thus both are depicted. Please refer toSupplementary Data 2 and 3for complete depiction of our analysis with and without the inclusion of leukocyte-associated genes. The normal lung circadian transcriptome In healthy lungs, 1,067 genes (1,190 probes) exhibited reproducible rhythmic expression ( Supplementary Data 1 ), and 321 of these genes were uniquely rhythmic in mouse lung ( Supplementary Table 1 ). To gain insight into the functions of these circadian-regulated genes we performed functional annotation analysis, using enrichment P -value as a means of ranking. Twenty Kyoto Encyclopedia of Genes and Genomics (KEGG) pathway terms achieved our threshold for enrichment (cutoff P <0.05), and could be temporally segregated into two loose clusters positioned at subjective mid-day and late night ( Fig. 1 and Supplementary Data 2 ). Interestingly, the majority of KEGG terms enriched in the mid-day cluster were related to immune function, and 158/1,067 genes overall (14.8%) had a leukocyte-related annotation (red-highlighted terms in Fig. 1 ). In contrast, KEGG terms related to mitotic signalling were segregated to the later half of the dark phase and were largely independent of immune-related pathways, as exclusion of the 158 leukocyte-associated genes did not abrogate their functional enrichment ( Fig. 1 and Supplementary Data 3 ). Our prevailing impression from this analysis was that immune processes are heavily represented in the circadian transcriptome of healthy mouse lungs, a finding not emphasized in published meta-analyses of other mouse solid organs [6] . As a result, mouse lung represented an opportune setting to examine how inflammation affects organ-wide circadian regulation. Figure 1: Temporal map of KEGG terms enriched in the basal circadian transcriptome of mouse lung. The 4-h phase interval that returned the lowest enrichment P -value (EASE score modification of the Fisher exact test [61] ) for a given KEGG term was used to position that term on the map. Time of day is expressed in ‘CT’, with CT0 representing the beginning of the light phase and CT12 the beginning of the dark phase. Terms that were also enriched in the master list of 1,190 probes (without consideration of acrophase) are bolded and in caps. Terms whose enrichment at P <0.05 depended on the inclusion of leukocyte-associated genes (see Methods) are coloured red. For clarity, only terms with enrichment P -values <0.01 are depicted. Note for two KEGG Terms (Circadian Rhythm and Systemic Lupus Erythemasosis), there were two optima in P -values in the basal state and thus both are depicted. Please refer to Supplementary Data 2 and 3 for complete depiction of our analysis with and without the inclusion of leukocyte-associated genes. Full size image Endotoxemia reprogrammes lung circadian gene expression To examine how systemic inflammation affects lung circadian rhythms, we challenged mice with a single intraperitoneal injection of Escherichia coli endotoxin sufficient to produce >80% mortality by 3 days ( Supplementary Fig. 2 ). In mouse lung, endotoxin disrupted the circadian expression of core molecular clock genes, with some becoming arrhythmic and others showing a distorted but rhythmic pattern compared with baseline ( Fig. 2a and Supplementary Data 4 ). However, at the genome-wide scale, circadian gene expression was not globally suppressed. Of the 1,190 probes that exhibited reproducible circadian regulation in the healthy state, 668 retained evidence of rhythmic expression according to our analytical protocol (see Methods) and 291 (24.4%) retained period lengths within a general circadian range of 15–36 h per cycle ( Supplementary Data 1 ). At the same time, endotoxemia induced rhythmic expression in 5,121 new genes (5,952 probes) that were not identified as basally circadian regulated in the lung in either microarray experiment ( Supplementary Data 5 ). Of these, 2,241 genes (2,517 probes) exhibited circadian–range period lengths of 15–36 h and 963 genes were unique to mouse lung ( Supplementary Table 1 ). Taken together, circadian patterns of gene expression were at least as common in the lung during endotoxemia as in the basal state, and encompassed a largely divergent set of genes ( Fig. 2b ). Functional annotation analysis of the endotoxin-specific circadian transcriptome indicated continued enrichment for immune-related processes during endotoxemia ( Fig. 3 and Supplementary Data 6 ). However, the particular KEGG terms enriched during endotoxemia were different and included pathways governing the response to ‘pathogen-associated molecular patterns’ (PAMPs) [13] . Of note 250/2,241 genes (11.1%) had leukocyte-associated annotations and accounted for the enrichment of most (but not all) PAMP-related KEGG terms ( Fig. 3 and Supplementary Data 6 and 7 ). To summarize, lung circadian gene expression persisted at a genome-wide scale during endotoxemia despite clock gene disruptions and was shifted to a largely new set of genes and immunologic processes. 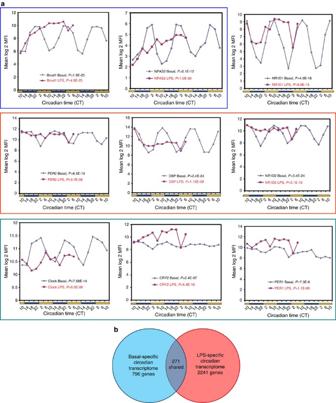Figure 2: Endotoxemia alters clock gene expression patterns and the composition of the lung circadian transcriptome. (a) Expression patterns of core circadian clock genes in mouse lung during the basal state (blue line) and endotoxemia (red line). Each data point represents the mean Log2MFI (n=3–4 mice) derived from Microarray Experiment 2, which were housed under constant light (LL 12:12) conditions. Statistical significance as determined via one-way ANOVA is depicted. Genes exhibiting qualitatively similar expression patterns during endotoxemia are enclosed together in coloured rectangles (monotonic induction of expression (bmal1,npas2; blue rectangle), depression of circadian amplitude (per2,dbp,nr1d2; red rectangle) and retention of rhythmic expression but with an altered pattern (clock,cry2,per1; green rectangle)). Probe identifications and rhythm analysis for these data are listed inSupplementary Data 4. (b) Venn diagram depicting the extent of overlap between the basal and endotoxin-associated circadian transcriptome. Figure 2: Endotoxemia alters clock gene expression patterns and the composition of the lung circadian transcriptome. ( a ) Expression patterns of core circadian clock genes in mouse lung during the basal state (blue line) and endotoxemia (red line). Each data point represents the mean Log 2 MFI ( n =3–4 mice) derived from Microarray Experiment 2, which were housed under constant light (LL 12:12) conditions. Statistical significance as determined via one-way ANOVA is depicted. Genes exhibiting qualitatively similar expression patterns during endotoxemia are enclosed together in coloured rectangles (monotonic induction of expression ( bmal1 , npas2 ; blue rectangle), depression of circadian amplitude ( per2 , dbp , nr1d2 ; red rectangle) and retention of rhythmic expression but with an altered pattern ( clock , cry2 , per1 ; green rectangle)). Probe identifications and rhythm analysis for these data are listed in Supplementary Data 4 . ( b ) Venn diagram depicting the extent of overlap between the basal and endotoxin-associated circadian transcriptome. 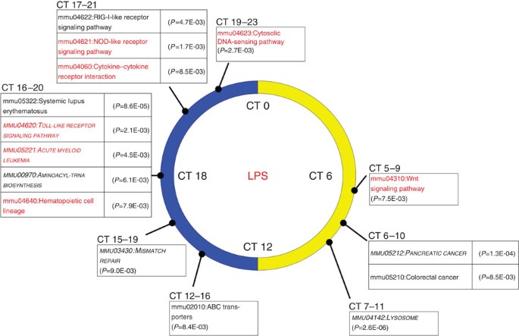Figure 3: Temporal map of KEGG terms enriched in endotoxemia-specific circadian transcriptome of mouse lung. The 4-h phase interval that returned the lowest enrichmentP-value (EASE score modification of the Fisher exact test61) for a given KEGG term was used to position that term on the map. Terms that were also enriched in the master list of 2,517 probes (without consideration of acrophase) are bolded and in caps. Terms whose enrichment atP<0.05 depended on the inclusion of leukocyte-associated genes (see Methods) are coloured red. For clarity, only terms with enrichmentP-values <0.01 are depicted. Please refer toSupplementary Data 6 and 7for complete depiction of our analysis with and without the inclusion of leukocyte-associated genes. Full size image Figure 3: Temporal map of KEGG terms enriched in endotoxemia-specific circadian transcriptome of mouse lung. The 4-h phase interval that returned the lowest enrichment P -value (EASE score modification of the Fisher exact test [61] ) for a given KEGG term was used to position that term on the map. Terms that were also enriched in the master list of 2,517 probes (without consideration of acrophase) are bolded and in caps. Terms whose enrichment at P <0.05 depended on the inclusion of leukocyte-associated genes (see Methods) are coloured red. For clarity, only terms with enrichment P -values <0.01 are depicted. Please refer to Supplementary Data 6 and 7 for complete depiction of our analysis with and without the inclusion of leukocyte-associated genes. Full size image Endotoxin alters circadian gene expression periodicity To better understand how circadian gene expression is organized during lung inflammation, we examined how endotoxin had an impact on the distributions of key parameters used to define circadian rhythms (mesor, amplitude, period and acrophase; see Methods) [14] . We focused first on the 1,190 probes that constituted the normal lung circadian transcriptome. Although endotoxin did not shift the mesor (mean abundance) or amplitude of these rhythmically regulated probes on a population level ( Supplementary Fig. 3 ), it strongly affected the periodicity of gene expression ( Fig. 4 ). Rather than a single cluster at the expected circadian period duration of 24–25 h, endotoxin shifted the distribution to 3 clusters at 9 h (92 probes), 20 h (232 probes) and >47 h (193 probes; Fig. 4a,b,e ). Of probes that exhibited circadian–range periodic expression (15–36 h), endotoxin shifted period lengths from a median of 25.4 h to 19.6 h ( P =2.8E−11, paired 2-tailed t -test of log 2 -transformed data, n =291). Endotoxin also affected the distribution of acrophases in the circadian transcriptome. In the basal state, acrophases exhibited a unimodal distribution centred in the early subjective day ( Fig. 4c,d,e ), similar to observations in other organs [15] . However, endotoxin eliminated this clustering of acrophases and, for the subset of probes that retained circadian–range periods of 15–36 h, induced a bimodal distribution ( Fig. 4c,d,e ). We next focused on the endotoxin-specific circadian transcriptome and found these genes also exhibited identically shortened period lengths and bimodal acrophase distributions ( Supplementary Fig. 4 ). We concluded that endotoxemia not only changed the identities of genes engaged in circadian variation but also manipulated their periodicity and phase to produce a distinctive temporal organization. Moreover, the oscillatory signature produced by endotoxin predominated over that of the normal molecular clock. 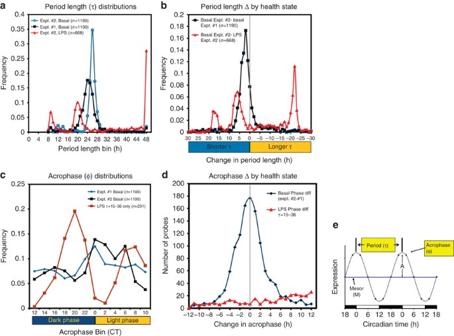Figure 4: Endotoxemia regulates circadian period length and acrophase. (a) Histogram depicting the distribution of period lengths (τ) for the microarray probes exhibiting significant rhythmic oscillations in normal mouse lung (n=1,190) and endotoxemia (n=668). The black and blue lines represent data from the basal groups of Microarray Experiments 1 and 2, respectively. The red line represents period lengths from the endotoxemia group of Microarray Experiment 2. (b) Histogram depicting changes in period length for individual probes, comparing the basal state in two independent microarray experiments (reflective of inter-experimental variability) versus changes as a result of endotoxemia. The black line represents period length differences between basal groups of Microarray Experiments 1 and 2 (n=1,190). The red line represents period length differences between basal and endotoxemia groups of Microarray Experiment 2 (n=668). (c) Histogram depicting the distribution of acrophases (φ) for the lung circadian transcriptome in the basal state versus endotoxemia. The blue and black lines represent data from the control groups of Microarray Experiments 1 and 2, respectively (n=1,190). The red line represents acrophases during endotoxemia in Microarray Experiment 2 for probes whose period lengths were of circadian-like duration (between 15 and 36 h (n=291)). (d) Histogram of acrophase differences for individual probes. The black line represents acrophase differences between the basal groups of Microarray Experiments 1 and 2 (n=1,190). The red line represents acrophase differences between the basal and endotoxemia groups of Microarray Experiment 2 (n=291). (e) Schematic of an idealized waveform with the circadian rhythm characteristics of period and acrophase highlighted in yellow. Figure 4: Endotoxemia regulates circadian period length and acrophase. ( a ) Histogram depicting the distribution of period lengths ( τ ) for the microarray probes exhibiting significant rhythmic oscillations in normal mouse lung ( n =1,190) and endotoxemia ( n =668). The black and blue lines represent data from the basal groups of Microarray Experiments 1 and 2, respectively. The red line represents period lengths from the endotoxemia group of Microarray Experiment 2. ( b ) Histogram depicting changes in period length for individual probes, comparing the basal state in two independent microarray experiments (reflective of inter-experimental variability) versus changes as a result of endotoxemia. The black line represents period length differences between basal groups of Microarray Experiments 1 and 2 ( n =1,190). The red line represents period length differences between basal and endotoxemia groups of Microarray Experiment 2 ( n =668). ( c ) Histogram depicting the distribution of acrophases ( φ ) for the lung circadian transcriptome in the basal state versus endotoxemia. The blue and black lines represent data from the control groups of Microarray Experiments 1 and 2, respectively ( n =1,190). The red line represents acrophases during endotoxemia in Microarray Experiment 2 for probes whose period lengths were of circadian-like duration (between 15 and 36 h ( n =291)). ( d ) Histogram of acrophase differences for individual probes. The black line represents acrophase differences between the basal groups of Microarray Experiments 1 and 2 ( n =1,190). The red line represents acrophase differences between the basal and endotoxemia groups of Microarray Experiment 2 ( n =291). ( e ) Schematic of an idealized waveform with the circadian rhythm characteristics of period and acrophase highlighted in yellow. Full size image Endotoxin alters leukocyte circadian rhythms in the lung Given the prominence of leukocyte-associated genes in both the normal and endotoxin-associated circadian transcriptome, we investigated whether there were temporal variations in leukocyte abundance in mouse lung that could have an impact on the gene expression data. Using flow cytometry, we detected a 2.3-fold circadian variation in the number of CD45 + cells in the lungs of healthy mice but not in the spleens of the same animals ( Fig. 5a,b ). This time effect required an intact circadian clock, as bmal1 -null mice, which lack a functional circadian clock [16] , did not exhibit temporal variation in CD45 + cell number ( Fig. 5c ). Similarly, B cells (CD45 + -CD19 + ), but not T cells, were temporally regulated ( Supplementary Fig. 5 ). Interestingly, oscillations in the B-cell marker CD19 were driven primarily by variations in B-cell number in the lung, rather than cell-intrinsic oscillations in CD19 protein levels ( Supplementary Fig. 6 ). In contrast, some genes specific to leukocytes, such as fas , had expression patterns in anti-phase to CD45 + and CD19 + cell numbers ( Supplementary Data 1 ). Taken together, oscillations in cell counts could explain the circadian expression of many but not all leukocyte-related genes. 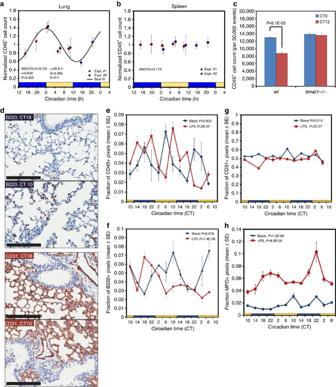Figure 5: Circadian variation in mouse lung leukocytes in the basal state and endotoxemia. Flow cytometric measurement of CD45+cell number normalized to the time-averaged mean from dissociated whole lungs (a) and spleens (b). SeeSupplementary Fig. 10for representative gates. Data points represent the mean±s.e. (n=4–6 mice). Data from two independent time-series experiments are aligned on the time coordinate (expressed in units of CT). Statistical significance (via one-way ANOVA) and best-fit rhythm parameters are depicted where appropriate. The estimated best-fit cosine curve (black line) is also plotted. (c) Circadian variation in CD45+cell counts inbmal1-null andwtlungs. Data represent the mean ofn=5 mice±s.e. Statistical significance was determined by two-tailedt-test. (d) Representative IHC depicting B220+B-cell number at two time points (representing the peak and nadir of abundance), as well as CD31+endothelial cells (coloured orange). Scale bar, 200 μm. (e–h) Leukocyte rhythms in the mouse lung as measured by IHC. Blue lines represent positive pixel counts from healthy lungs and red lines represent endotoxemic lungs. Each point represents the mean normalized positive pixel count±s.e. (n=2–3). (e) CD45 staining. (f) B220 staining. (g) CD31 staining. (h) MPO staining. Statistical significance via one-way ANOVA is depicted in the legends. The results depicted represent positive pixel counts of at least moderate intensity as specified by the commercial algorithm (see Methods), but results were similar using both higher and lower thresholds (seeSupplementary Data 8for tabular presentation of these data). Note that mice used for flow cytometry experiments (a–c) were housed under constant dark (DD 12:12) conditions and mice used for IHC (d–h) derived from Microarray Experiment 2 and were housed under constant light (LL 12:12 conditions). Figure 5: Circadian variation in mouse lung leukocytes in the basal state and endotoxemia. Flow cytometric measurement of CD45 + cell number normalized to the time-averaged mean from dissociated whole lungs ( a ) and spleens ( b ). See Supplementary Fig. 10 for representative gates. Data points represent the mean±s.e. ( n =4–6 mice). Data from two independent time-series experiments are aligned on the time coordinate (expressed in units of CT). Statistical significance (via one-way ANOVA) and best-fit rhythm parameters are depicted where appropriate. The estimated best-fit cosine curve (black line) is also plotted. ( c ) Circadian variation in CD45 + cell counts in bmal1 -null and wt lungs. Data represent the mean of n =5 mice±s.e. Statistical significance was determined by two-tailed t -test. ( d ) Representative IHC depicting B220 + B-cell number at two time points (representing the peak and nadir of abundance), as well as CD31 + endothelial cells (coloured orange). Scale bar, 200 μm. ( e – h ) Leukocyte rhythms in the mouse lung as measured by IHC. Blue lines represent positive pixel counts from healthy lungs and red lines represent endotoxemic lungs. Each point represents the mean normalized positive pixel count±s.e. ( n =2–3). ( e ) CD45 staining. ( f ) B220 staining. ( g ) CD31 staining. ( h ) MPO staining. Statistical significance via one-way ANOVA is depicted in the legends. The results depicted represent positive pixel counts of at least moderate intensity as specified by the commercial algorithm (see Methods), but results were similar using both higher and lower thresholds (see Supplementary Data 8 for tabular presentation of these data). Note that mice used for flow cytometry experiments ( a – c ) were housed under constant dark (DD 12:12) conditions and mice used for IHC ( d – h ) derived from Microarray Experiment 2 and were housed under constant light (LL 12:12 conditions). Full size image In contrast to other leukocyte types, alveolar macrophages (CD45 + -CD11c + -Siglec-F + ) exhibited a low amplitude rhythm that was inverted relative to the CD45 + population as a whole ( Supplementary Fig. 7a ). The highest amplitude circadian effect among the subtypes tested was the CD45 + -CD11b + -Gr1 + granulocyte population ( Supplementary Fig. 7c ). Lung epithelial cells (CD45 − -EPCAM + ), endothelial cells (CD45 − -CD31 + ) and monocytes (CD45 + -CD11b + -GR1 − ) did not exhibit significant temporal variation in mouse lung ( Supplementary Fig. 7d,e,b ). Using IHC as an alternative means of quantifying leukocyte number (see Methods), we confirmed that CD45 + leukocyte and B220 + B-cell counts oscillate in healthy mouse lungs ( Fig. 5d–f and Supplementary Data 8 ). In contrast, CD31 + endothelial cell counts did not oscillate ( Fig. 5g ). During endotoxemia, we found that MPO + granulocyte number exhibited circadian-like variation in the lung ( Fig. 5h and Supplementary Data 8 ). In contrast, rhythmic variation in B cells was dampened, while endothelial cell staining was not grossly affected ( Fig. 5f,g ). Total haematopoietic (CD45 + ) cell counts retained evidence of rhythmic abundance in either health state; however, the temporal pattern was altered by endotoxemia and became less regular ( Fig. 5e ). Taken together, endotoxemia re-organized circadian patterns of leukocyte abundance in mouse lung away from B-cell rhythms and towards MPO + granulocytes. Leukocyte rhythms partially accounted for the immunologic character of the lung circadian transcriptome in either health state. Endotoxin reprogrammes the lung circadian metabolome Besides messenger RNA, circadian rhythms regulate the abundance of other kinds of biomolecules, including low-molecular weight metabolites [17] , [18] . As metabolite circadian rhythms and clock gene expression patterns are thought to reinforce one another through feedback regulation [19] , [20] , [21] , we examined the lung circadian metabolome using a well-established commercial panel [22] . Our question was whether endotoxin produced a reprogramming of the lung circadian metabolome similar to the circadian transcriptome. Under basal conditions, we identified 50 metabolites that exhibited rhythmic variation in mouse lung ( Supplementary Data 9 ). As expected, the periodicity of rhythmic metabolites in the basal state clustered in a single peak at 24–25 h similar to the circadian transcriptome ( Fig. 6a ). In addition, the distribution of metabolite acrophases assumed a unimodal cluster similar to normal circadian gene expression, although the peak for metabolites was offset 6 h into the dark phase relative to the transcriptome ( Fig. 6b ). 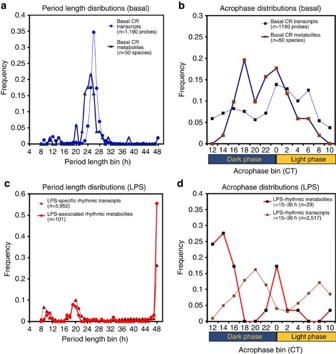Figure 6: The lung circadian transcriptome and metabolome exhibit temporal coupling during endotoxemia. (a) Period length distributions for the basal lung circadian metabolome (thick blue line, closed triangles) and transcriptome (thin blue line, closed circles). (b) Histogram comparison of acrophases for the basal lung circadian metabolome (thick blue line, closed orange squares) and transcriptome (thin blue line, closed black squares). (c) Histogram comparison of period lengths during endotoxemia for rhythmic metabolites (red line, closed circles) and rhythmic gene expression (brown line, closed triangles). (d) Histogram comparison of acrophases during endotoxemia for rhythmic metabolites (red line, black squares) and rhythmic gene expression (brown, brown squares). For clarity, only metabolites and probes exhibiting periods of 15–36 h are depicted. All biological samples were obtained from mice used for Microarray Experiment 2. Figure 6: The lung circadian transcriptome and metabolome exhibit temporal coupling during endotoxemia. ( a ) Period length distributions for the basal lung circadian metabolome (thick blue line, closed triangles) and transcriptome (thin blue line, closed circles). ( b ) Histogram comparison of acrophases for the basal lung circadian metabolome (thick blue line, closed orange squares) and transcriptome (thin blue line, closed black squares). ( c ) Histogram comparison of period lengths during endotoxemia for rhythmic metabolites (red line, closed circles) and rhythmic gene expression (brown line, closed triangles). ( d ) Histogram comparison of acrophases during endotoxemia for rhythmic metabolites (red line, black squares) and rhythmic gene expression (brown, brown squares). For clarity, only metabolites and probes exhibiting periods of 15–36 h are depicted. All biological samples were obtained from mice used for Microarray Experiment 2. Full size image Endotoxin produced extensive changes to the temporal expression of circadian metabolites ( Fig. 7 and Supplementary Data 9 and 10 ), including disruption of oscillations (32/50 metabolites), and induction of new circadian rhythms (21 novel metabolites with period durations 15–36 h). Endotoxin shifted the period-length distribution of metabolites from a single peak at 24–25 h to three peaks at 9, 20 and >47 h ( Fig. 6c ). The acrophase distribution for metabolites shifted with endotoxin from a unimodal to a bimodal distribution but, interestingly, the 6-h offset between metabolite and transcript acrophases was retained ( Fig. 6d ). Most strikingly, endotoxin affected the period and acrophase distributions of the circadian metabolome in a nearly identical manner to that of the circadian transcriptome. Our findings demonstrate that at a genome-wide scale, the circadian transcriptome and metabolome are temporally coupled during endotoxemia despite disruptions to clock gene expression. Our results further imply that a shared system of regulation links circadian gene and metabolite expression during endotoxemia, and that this system does not require normal gene expression relationships between canonical clock genes to function. 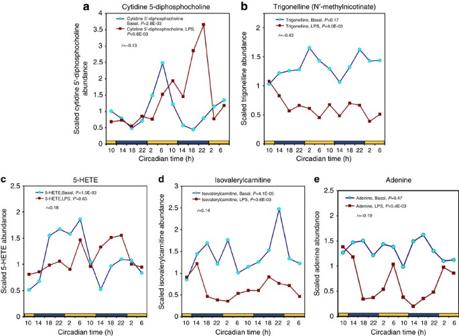Figure 7: Representative metabolite abundances over time meant to illustrate the diverse effects of endotoxemia on the lung circadian metabolome. Each data point represents the mean metabolite abundance (n=3) scaled to the median (see Methods). Statistical significance via one-way ANOVA and Pearson’srvalues comparing basal with endotoxemic lungs are depicted. (a) Cytidine 5′-diphosphocholine. (b) Trigonelline. (c) 5-HETE. (d) Isovalerylcarnitine. (e) Adenine. Figure 7: Representative metabolite abundances over time meant to illustrate the diverse effects of endotoxemia on the lung circadian metabolome. Each data point represents the mean metabolite abundance ( n =3) scaled to the median (see Methods). Statistical significance via one-way ANOVA and Pearson’s r values comparing basal with endotoxemic lungs are depicted. ( a ) Cytidine 5′-diphosphocholine. ( b ) Trigonelline. ( c ) 5-HETE. ( d ) Isovalerylcarnitine. ( e ) Adenine. Full size image Although the feedback relationships between metabolites and circadian gene expression are incompletely understood, a handful of metabolite-sensing pathways, including NAD + /Sirt1 (refs 19 , 21 ), AMPK [23] and mTORC1 (ref. 24 ) have been shown to affect clock gene expression. We therefore analysed the effects of endotoxin on markers of these pathways in mouse lung. In healthy lungs, both NAD + and NADP + nucleotides exhibited ultradian variations in abundance and these were blunted by endotoxin ( Fig. 8a,b and Supplementary Data 11 ). RS6 phosphorylation, reflective of mTORC1 activity, exhibited low-amplitude circadian variations in the healthy lungs ( Fig. 8c, d and Supplementary Data 11 ). During endotoxemia, overall rS6 phosphorylation was increased but circadian variation in this marker was disrupted ( Fig. 8c,d and Supplementary Data 11 ). Variations in AMPKα phosphorylation were also altered in the endotoxemic lung ( Fig. 8c,e and Supplementary Data 11 ). Our results suggest that endotoxin disrupts the normal activity patterns of metabolite-sensing pathways known to affect clock gene expression. However, by themselves disruptions to these pathways do not clearly explain the phenomenon of endotoxin-associated circadian rhythms within the lung. 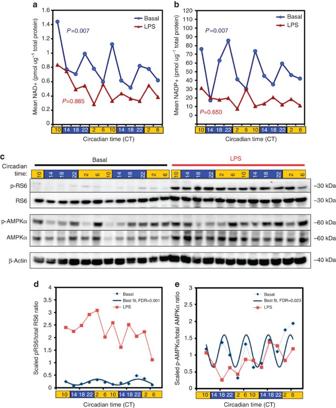Figure 8: Effect of lung endotoxemia on metabolite-sensing pathways known to regulate clock gene expression patterns. Lung homogenates used for these measurements were derived from Microarray Experiment 2. Mean levels of NAD+(a) and NADP+nucleotides (b) in basal and endotoxemic lungs. Each point represents data obtained from pooled lung homogenates (n=3). Blue lines represent lungs from PBS-treated animals and red lines represent lungs from endotoxemic animals. Significance values for each curve are depicted (ANOVA periodogram assumingτ=12 h). (c) Western blot analysis of phospho-rS6 (Ser 235/236) and phospho-AMPKα1/2 (Thr 172) abundance over time in normal and endotoxemic lungs. Each lane represents 25 μg total protein pooled fromn=3 lungs. Similar results were obtained in two independent time-series experiments. Densitometric measurement of phsopho-rS6/total rS6 ratio (d) and phospho-AMPKα total AMPKα ratio (e). Blue lines represent data from normal lungs and red lines represent data from endotoxemic lungs. A best-fit single harmonic cosine curve is depicted where appropriate. For tabular depiction of COSOPT rhythm analyses of NAD+levels, NADP+levels, phsopho-rS6/total rS6 ratio and phospho-AMPKα total AMPKα ratio please seeSupplementary Data 11. Full images of the western blottings are depicted inSupplementary Fig. 12. Note that for these experiments, data were collected under constant light (LL 12:12) conditions. Figure 8: Effect of lung endotoxemia on metabolite-sensing pathways known to regulate clock gene expression patterns. Lung homogenates used for these measurements were derived from Microarray Experiment 2. Mean levels of NAD + ( a ) and NADP + nucleotides ( b ) in basal and endotoxemic lungs. Each point represents data obtained from pooled lung homogenates ( n =3). Blue lines represent lungs from PBS-treated animals and red lines represent lungs from endotoxemic animals. Significance values for each curve are depicted (ANOVA periodogram assuming τ =12 h). ( c ) Western blot analysis of phospho-rS6 (Ser 235/236) and phospho-AMPKα1/2 (Thr 172) abundance over time in normal and endotoxemic lungs. Each lane represents 25 μg total protein pooled from n =3 lungs. Similar results were obtained in two independent time-series experiments. Densitometric measurement of phsopho-rS6/total rS6 ratio ( d ) and phospho-AMPKα total AMPKα ratio ( e ). Blue lines represent data from normal lungs and red lines represent data from endotoxemic lungs. A best-fit single harmonic cosine curve is depicted where appropriate. For tabular depiction of COSOPT rhythm analyses of NAD + levels, NADP + levels, phsopho-rS6/total rS6 ratio and phospho-AMPKα total AMPKα ratio please see Supplementary Data 11 . Full images of the western blottings are depicted in Supplementary Fig. 12 . Note that for these experiments, data were collected under constant light (LL 12:12) conditions. Full size image Given that the circadian transcriptome and metabolome appear temporally coupled during endotoxemia, we asked whether circadian rhythms in gene expression and metabolites could jointly produce effects that are relevant to lung inflammation. Using joint functional enrichment analysis (see Methods), we identified purine metabolism as temporally regulated in both health states at both the mRNA and metabolite level ( Supplementary Data 12 and 13 ). We focused on urate, an inflammatory mediator that is the terminal product of purine metabolism [25] , and found that during endotoxemia there was rhythmic accumulation of this metabolite in the lung ( Fig. 9a ). Interestingly, urate was recently identified as a physiological substrate for MPO that catalyses its conversion to allantoin [26] . Given our observation that granulocytes rhythmically infiltrate the lung during endotoxemia, we compared the expression patterns of mpo and urate under endotoxemia and observed a clear reciprocal relationship ( Fig. 9b ). Moreover, allantoin, a breakdown product of urate [25] , accumulated in direct proportion to mpo expression as well as MPO + granulocyte number ( Fig. 9b,c ). Urate is significant because elevated amounts can lead to the formation of uric acid crystals that stimulate interleukin-1β release from macrophages via the Nlrp3 inflammasome [27] . Of note, nlrp3 expression developed temporal variation in the setting of endotoxin that paralleled the expression pattern of urate ( Fig. 9d ). To summarize, endotoxin promoted temporal oscillations in urate levels probably through the rhythmic infiltration of MPO + granulocytes into the lung, resulting in synchronization with nlrp3 expression. This illustrates how cellular and molecular circadian rhythms can synergize in the endotoxemic lung and jointly impact urate signalling, a pathway germane to lung inflammation [28] , [29] . It also indicates a level of systems integration usually associated with homeostatic circadian rhythms in healthy organisms [1] . 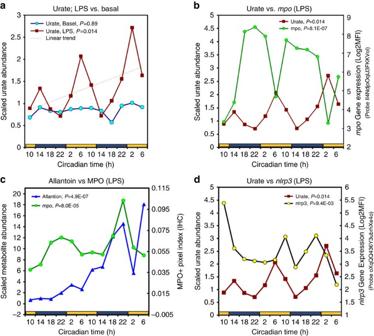Figure 9: Temporal regulation of uric acid metabolism during endotoxemia. Each point represents the mean (n=3). Statistical significance via one-way ANOVA is depicted in the legends. (a) Urate level in the basal (blue line) and endotoxemic states (red line). For endotoxemic lung, the linear trend is depicted as a dotted line. (b) Urate level (red line) versusmpoexpression (green line). (c) Allantoin level (blue line) versus MPO+granulocyte abundance in endotoxemic lungs (green line). (d) Urate level versusnrlp3expression (black line). Note that mice used for these experiments were derived from Microarray Experiment 2 and were housed under constant light (LL 12:12) conditions. Figure 9: Temporal regulation of uric acid metabolism during endotoxemia. Each point represents the mean ( n =3). Statistical significance via one-way ANOVA is depicted in the legends. ( a ) Urate level in the basal (blue line) and endotoxemic states (red line). For endotoxemic lung, the linear trend is depicted as a dotted line. ( b ) Urate level (red line) versus mpo expression (green line). ( c ) Allantoin level (blue line) versus MPO + granulocyte abundance in endotoxemic lungs (green line). ( d ) Urate level versus nrlp3 expression (black line). Note that mice used for these experiments were derived from Microarray Experiment 2 and were housed under constant light (LL 12:12) conditions. Full size image Granulocyte rhythms in inflamed lungs are bmal1 dependent To examine whether the endotoxin-specific circadian programme shares mechanistic elements with the normal molecular clock, we subjected bmal1 -null mice to endotoxemia. Interestingly, bmal1 deficiency did not greatly affect the rhythmic expression of cldn2 and ace during endotoxemia ( Fig. 10a,b ), genes whose expression is normally specific to epithelial cells [30] and endothelial cells [31] , respectively. However, the temporal expression of leukocyte-associated genes ifn γ and mpo was significantly altered in lungs of endotoxemic bmal1 -null mice compared with wt ( Fig. 10c,d ). In the case of ifn γ, the expression pattern was more variable in bmal1 -null animals such that it failed to achieve statistical significance by one-way analysis of variance (ANOVA), while for mpo expression the amplitude of the rhythm was reduced. As ifn γ and mpo expression are both highly expressed by granulocytes, we analysed granulocyte counts in endotoxemic lungs via IHC. Although the mesor for MPO + granulocyte counts was similar in bmal1 -null mice and wt mice after endotoxin, the circadian pattern of MPO + cell number was lost in bmal1 -deficient lungs ( Fig. 10e,f and Supplementary Data 14 ). To further understand why bmal1 deletion might affect rhythmic gene expression in a differential manner, we examined the pattern of bmal1 expression in mouse lung using IHC ( Supplementary Fig. 8 ). Similar to previous observations [32] , we found that bmal1 expression was not ubiquitous in the lung but rather was concentrated in airway epithelial cells and scattered cells in the alveolar space, the distribution of which was consistent with leukocytes and type II pneumocytes ( Supplementary Fig. 8a ). Staining of type I pneumocytes and endothelial cells, the predominant structural cells in the alveolar space [33] , was not apparent. Finally, endotoxemia did not grossly shift the histological pattern of lung bmal1 expression ( Supplementary Fig. 8b ). Taken together, our data suggest that bmal1 selectively contributes to circadian regulation in the endotoxemic lung: being important for rhythmic granulocyte recruitment and gene expression but less important for gene expression rhythms in structural lung cells. This might be explained in part by the differential expression of bmal1 in mouse lung. 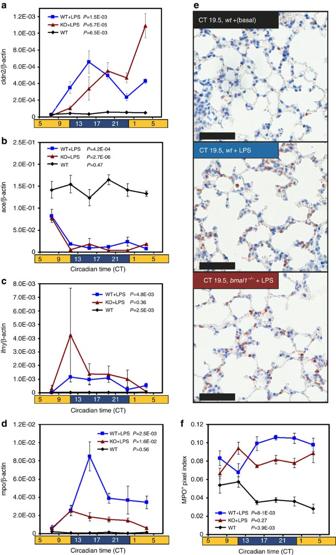Figure 10:Bmal1deficiency has selective effects on lung circadian gene expression and granulocyte trafficking during endotoxemia. Quantitative PCR analysis ofcldn2(a),ace(b),ifn-γ (c) andmpo(d) gene expression. Each data point represents mean expression normalized toβ-actin±s.e. (n=3–4). Significance values via one-way ANOVA are depicted within each graph. Red lines represent lungs frombmal1-null mice treated with 10 mg kg−1endotoxin intraperitoneal (i.p.) directly before the first time point and kept under constant light (LL 12:12) conditions. Blue lines represent lungs from endotoxemicwtlittermates and black lines represent lungs from untreatedwtmice. For ease of comparison, corresponding expression data from Microarray Experiment 2 is shown inSupplementary Fig. 11. (e) Representative IHC depicting MPO+granulocyte counts at CT19.5. Scale bar, 60 μm. (f) MPO+granulocyte counts in mouse lung over time as measured by IHC. Each point represents the mean normalized positive pixel count±s.e. (n=3–4). Red lines represent endotoxemic lungs frombmal1-null mice, blue lines represent lungs from endotoxemicwtlittermates and black lines represent lungs from untreatedwtmice. Significance values via one-way ANOVA are depicted within each graph. The results depicted represent positive pixel counts of moderate intensity as specified by the commercial algorithm (see Methods). SeeSupplementary Data 14for COSOPT rhythm analysis of these data. Figure 10: Bmal1 deficiency has selective effects on lung circadian gene expression and granulocyte trafficking during endotoxemia. Quantitative PCR analysis of cldn2 ( a ), ace ( b ), ifn -γ ( c ) and mpo ( d ) gene expression. Each data point represents mean expression normalized to β-actin ±s.e. ( n =3–4). Significance values via one-way ANOVA are depicted within each graph. Red lines represent lungs from bmal1 -null mice treated with 10 mg kg −1 endotoxin intraperitoneal (i.p.) directly before the first time point and kept under constant light (LL 12:12) conditions. Blue lines represent lungs from endotoxemic wt littermates and black lines represent lungs from untreated wt mice. For ease of comparison, corresponding expression data from Microarray Experiment 2 is shown in Supplementary Fig. 11 . ( e ) Representative IHC depicting MPO + granulocyte counts at CT19.5. Scale bar, 60 μm. ( f ) MPO + granulocyte counts in mouse lung over time as measured by IHC. Each point represents the mean normalized positive pixel count±s.e. ( n =3–4). Red lines represent endotoxemic lungs from bmal1 -null mice, blue lines represent lungs from endotoxemic wt littermates and black lines represent lungs from untreated wt mice. Significance values via one-way ANOVA are depicted within each graph. The results depicted represent positive pixel counts of moderate intensity as specified by the commercial algorithm (see Methods). See Supplementary Data 14 for COSOPT rhythm analysis of these data. Full size image In this study we identified an alternate circadian regulatory programme that emerges in the endotoxemic lung despite disruptions to clock gene expression. Given that rhythmic clock gene expression is important for circadian rhythm generation in healthy mammals, one might have predicted that circadian regulation would be suppressed during endotoxemia. Instead, circadian-like rhythms proved to be widespread during endotoxemia at a genome-wide scale, observable at the level of transcripts, metabolites and leukocyte counts. Our results call into question the practice of using clock gene expression patterns as surrogate markers for circadian rhythms, a practice applied not just to inflammation but numerous other disorders, including lung models of cigarette smoke exposure [34] and ventilator injury [35] . Our data further distinguish the lung as a setting where circadian regulation of immune processes is easily observable. Although circadian fluctuations in leukocyte trafficking have been identified in other tissues [36] , [37] , [38] , [39] , immune processes were not previously reported to dominate functional enrichment analyses of circadian gene expression as they do in the lung. This may reflect the distinctive anatomy of the lung peripheral clock: unlike other organs where clock gene expression is ubiquitous, in the lung it is restricted to small airway epithelial cells and scattered cells in the alveoli [32] , a great many of which are probably leukocytes. Moreover, a large proportion of nucleated cells in the mammalian lung are of haematopoietic origin [33] , and presumably can influence the results of functional enrichment analyses by sheer force of numbers. This is not to imply that immune cells are devoid of intrinsic molecular clocks; indeed, clock gene expression was shown to be rhythmic in isolated B cells and peritoneal macrophages [40] , [41] . Rather, our data show there is an additional layer of circadian immune regulation within the lung at the level of cell number that must be taken into account if transcriptional profiling studies in the respiratory system are to be properly interpreted. When one considers the multiple pathways by which immune gene expression can achieve circadian variation in the lung, it is easy to see why circadian influences are prominent in normal airway physiology [12] , in common inflammatory diseases of the airway [11] , [42] , [43] , and as we show here during endotoxemia. Although lung anatomy may impart unique aspects to circadian regulation in the respiratory system, alternative circadian programming as a general concept may be present in other contexts. While this paper was under review, Eckel-Mahan et al . [44] identified clock-independent circadian rhythms in the livers of mice fed a high-fat diet. It may be that alternative circadian programming will prove a frequent feature of systemic disorders or disorders where whole-organ physiology is compromised. Further, it may be possible to subtype heterogeneous clinical entities, for example, acute lung injury, on the basis of their genome-wide circadian programmes. In healthy organisms, circadian rhythms serve to adjust the magnitude of inflammation in response to a given infectious stimulus [45] . However, little is known about what happens to circadian regulation at the molecular level in critically ill organisms. Current theory would hold that once an organism becomes acutely ill, circadian rhythms are disrupted and, beyond their absence, do not contribute further to pathogenesis [7] , [8] , [9] . However, our data shows that granulocyte influx into the endotoxemic lung has a strong circadian rhythmic component, and that this rhythm ‘sculpts’ both the accumulation of danger signals (such as urate) and the ability of the lung to respond to such signals (through the expression of PAMP-sensing pathways). Given that granulocyte recruitment to vital organs is a cardinal feature of the systemic inflammatory response, it would appear that circadian rhythms contribute fundamentally to how inflammation unfolds, at least in mouse lung. Are the endotoxin-associated rhythms we describe here truly ‘circadian’, or do they merely reflect negative feedback regulation unrelated to what is normally implied by this term? Formally, circadian rhythms are defined as 24-h cycles that are proved to be intrinsically generated and adjustable by environmental synchronizers such as food, light or temperature [46] . However, this formal definition is rarely fully applied in the literature when it comes to molecular and cellular circadian phenomena. For these kinds of microscopic rhythms, a more functional definition prevails: rhythms are circadian when they tie together disparate processes for the common end of streamlining daily physiologic activities. From this perspective, our data provide five lines of evidence to suggest endotoxin-associated rhythms are consistent with a circadian regulatory programme. First, roughly half of genes in the endotoxin-specific lung circadian transcriptome were also found to be circadian regulated in the basal state outside of the respiratory system ( Supplementary Table 1 ). Therefore, the endotoxin programme shares a kinship with circadian gene expression at the whole-organism level, although it is distinct from that of the healthy lung. Second, bmal1 , a prototypical molecular clock gene, was important for the circadian pattern of granulocyte infiltration into the endotoxemic lung. Third, the fact that endotoxin specifically altered period lengths and acrophases is significant, because changes to rhythmicity are the usual way circadian rhythms react to an entraining stimulus [47] . Fourth, oscillatory gene expression and metabolite abundance were temporally coupled during endotoxemia, an organizational feature in keeping with circadian regulation. Fifth, we found that during endotoxemia, rhythmic activity of leukocytes, transcripts and metabolites were integrated with each other and could coordinate pathways relevant to lung inflammation, as exemplified by the synchronized oscillations of urate abundance and nlrp3 expression. This kind of temporal orchestration, where a metabolite and a downstream mediator are synchronized, is characteristic of circadian function. For example, in normal liver, circadian regulation coordinates the expression of glycolytic enzymes to coincide with the anticipated time of glucose influx from food intake [48] . Taken together, the molecular and cellular rhythms that occur in the endotoxemic lung bear features consistent with a genuine circadian regulatory regime; albeit one that impacts inflammation rather than normal homeostasis. How are circadian-like rhythms generated in endotoxemic lungs despite the disrupted expression patterns of multiple clock genes and disrupted metabolic feedback pathways? One possibility is that the continued rhythmic expression of a subset of molecular clock genes (such as nr1d1 , per2 and cry2 ; Fig. 2a ) is sufficient to support an operational timekeeping mechanism, albeit one with different downstream effectors and different rhythmic properties. Another possibility is the circadian-like molecular rhythms we observed are products of a post-transcriptional clock similar to those described in bacteria and human erythrocytes [2] , [49] . We hope our data set will facilitate investigation of these questions, as well as examination of circadian contributions to immunologic function during respiratory diseases and systemic inflammation. Mice C57BL/6J male mice (4–6 weeks old, 20–25 g) were obtained from Jackson Laboratories and acclimatized for 2 weeks before use. We generated bmal1 -null mice by crossing Jackson Laboratory strains B6.129S4 (Cg)-Arntl tm1Weit /J and B6.C-Tg (CMV-cre)1Cgn/J. Heterozygote progeny where then mated to each other to obtain wild-type and bmal1 -null littermates as described [50] . Before all experiments, mice were fed a standard 20% protein rodent diet and housed in shoe box-type cages under a 12-h light/dark cycle. For all experiments, mice were euthanized with isofluorane and exsanguinated via direct cardiac puncture. All procedures performed on animals in this study were approved by the Harvard Medical School Institutional Review Board. Microarray experiment design To examine circadian regulation in mouse lung, we performed two independent time-series experiments (Microarray Experiments 1 and 2), in which groups of mice were euthanized at 4 h intervals for 48–72 h ( Supplementary Fig. 1a ). We varied light conditions and feeding conditions across the two experiments to control for known environmental cues that can affect circadian rhythm expression [51] . In one time-series experiment (Experiment 2), a subgroup of mice was subjected to endotoxemia, enabling us to compare the circadian transcriptome in the healthy versus the systemically inflamed state. For every probe that satisfied our rhythm detection protocol (see below), we represented the expression pattern in terms of four parameters typically used to define circadian rhythms ( Supplementary Fig. 1b ) [14] . These are as follows: mesor (M, the average level around which the rhythm varies), amplitude (A, the maximum deviation from the mesor), period length ( τ , the duration of each cycle and acrophase ( φ , the time at which expression is highest). We followed the standard convention of reporting times of day in units of CT, where CT0 represents lights-on and CT12 lights-off. In Microarray Experiment 1, 72 mice were segregated equally into 2 groups the day before the experiment at the beginning of the dark phase (CT12). In one group (LD 12:12), the mice were kept under standard lighting and nutritional conditions. In the second group (DD 12:12+STV), mice were kept in constant darkness and food pellets were removed from their cages at the start of sample acquisition. For Microarray Experiment 2, 94 mice were placed under constant light conditions (LL 12:12, food ad libitum ) at CT12 the day before. At CT10 on the day of the experiment, a subgroup of 40 mice received a single intraperitoneal injection of 12 mg kg −1 E. coli O127:B8 endotoxin (lipopolysaccharide (LPS), Sigma L3129, Lot 029K4055) and sample collection began directly after. For both Microarray Experiments 1 and 2, 3–4 mice per group were killed at consecutive 4-h intervals for 2–3 days ( Supplementary Fig. 1a ). The left lung and the right upper lobe were frozen immediately in liquid nitrogen for microarray and metabolomic analysis, and the right lower lobe was fixed by immersion in 2% paraformaldehyde. For mRNA isolation, lung tissue was immersed in RNAlater (Qiagen) and total RNA was then extracted using the RNeasy Mini Kit (Qiagen). RNA quality RNA Integrity Number (RIN) >7) was confirmed using an Agilent 2100 Bioanalyzer. RNA from all biological samples was labelled at once using the Ambion TotalPrep-96 RNA Amplification Kit. The samples were then blinded, randomized to chip position and hybridized to the Illumina MouseRef-8 v2.0 Expression BeadChips. For Microarray Experiment 1, RNA labelling and microarray hybridization were conducted at the Partners Center for Personalized Genetic Medicine, and for Microarray Experiment 2 at the Channing Division of Network Medicine (Brigham and Women’s Hospital). Resulting median fluorescence intensity (MFI) data were then normalized, log 2 -transformed, unmasked and then used for downstream analysis (see Supplementary Data 15–17 for normalized microarray data). In both Microarray Experiments 1 and 2, a single biological sample from each experiment (T4L2DD and T20L2, respectively) failed quality control and was excluded. Our sample sizes were chosen based on previously published analyses of circadian gene expression in various mouse and rat organs ( Supplementary Table 1 ). Data analysis Log 2 -transformed gene expression data was first pre-screened for probes, demonstrating statistically significant time-dependent variations by one-way ANOVA ( P -value cutoff <0.05) as described [51] . To identify probes that exhibit circadian variation, the data was next subjected to three different rhythm detection methods ( Supplementary Fig. 1a ). The first method (CYCLE) examined periodicity by computing a Fourier score (F) for each probe time series, reflecting its goodness-of-fit to a trigonometric function [52] : where i is the probe of interest, t is time and w =1 (for a 24-h circadian period). Significance was determined by computing Fourier scores for 100,000 random permutations of the probe time-series data. CYCLE data analysis was conducted using R Statistical software and the Cycle package of BioConductor 2.10 (available at http://www.bioconductor.org/packages/release/bioc/html/cycle.html ). The second method was autocorrelation [51] , which determined a correlation coefficient between the mean Log 2 MFI for the first six time points (covering the first 24 h of observation), versus time points 7–12 (the final 24 h of observation). Given a desired cutoff of P <0.05, we determined a cutoff value of r >0.73 based on the equation: where t is the t -distribution value (2.14 for this analysis given df=4, a one-tailed t -test and n =6). For the basal group of Microarray Experiment 2, there were 72 h of observation and, therefore, 3 possible comparisons between 24-h intervals. We selected the maximum r -value from the three possible comparisons to serve as the result for each probe. The third method was COSOPT [53] , [54] , which was written as a custom VBA macro in Microsoft Excel (available on request). For each probe, 9,576 cosine curves were generated using the equation: where i is the probe of interest, t is time in hours relative to the beginning of the experiment, M is the mesor (taken as the average of mean Log 2 MFI data for each probe), A is amplitude (taken as 1.5 times the s.d. of the mean Log 2 MFI values), τ is period length in hours (varied iteratively from 8 to 47.9 in 0.1-h steps) and φ is acrophase in hours (varied iteratively from 0 to 23.5 in 0.5-h steps). We were deliberately liberal in the range of period lengths examined to capture changes to the periodicity distribution as a result of endotoxemia, which would otherwise have been missed. The values for τ and φ (converted into units of CT) were reported from the cosine curve that among the 9,576 iterations produced the best goodness-of-fit to the mean time-series data (as measured by Pearson’s correlation coefficient ( r )). The optimal r -value was converted to a false detection rate (FDR) using a permutation test consisting of 1,000 random re-assortments of the time-series data (the period length was fixed at the value determined by COSOPT for the original data). The FDR was calculated as the number of permutations in which the r -value was equal or higher than that derived from the original data divided by 1,000. An FDR<0.05 was considered to represent a significant hit. For the purposes of this study, we regarded an expression pattern as rhythmic if it satisfied the ANOVA pre-screen and at least one rhythm detection method. If the expression pattern exhibited a period length between 15 and 36 h, we counted this as a circadian rhythm. Combined with a focus on reproducible rhythms in both microarray experiments, our analytical approach achieved 89% validation (8/9 genes tested), based on quantitative PCR analysis of independent time-series experiments ( Supplementary Figs 6a and 9 ). Functional annotation analysis We performed KEGG functional annotation enrichment analysis with DAVID 6.7 software (available at http://david.abcc.ncifcrf.gov/ ). We constructed a list of leukocyte-associated genes using available literature [55] , by searching mouse UNIPROT entries using the terms: ‘leukocyte, lymphocyte, neutrophil, monocyte, macrophage, dentritic, NK’, and by finding all genes on the microarray containing an annotation for ‘histocompatibility’ ( Supplementary Data 18 ). Co-enrichment of annotation terms in the microarray and metabolite data was examined using IMPaLA Software [56] (available at http://impala.molgen.mpg.de/ ). Quantitative real-time PCR Total RNA was isolated from lung homogenates using the RNeasy Mini Kit (Qiagen). Reverse transcription was carried out using the Applied Biosystems High Capacity cDNA Reverse Transcription Kit. Real-time PCR was performed on the ABI PRISM 7300 Sequence Detection System (Applied Biosystems) using TaqMan Gene Expression Master Mix (Applied Biosystems) and pre-designed TaqMan primers ( Supplementary Table 2 ). Relative ratios of mRNA were calculated using the 2 −ΔΔCt method with tbp or β-actin as the housekeeping gene. Statistical significance was tested by one-way ANOVA in Microsoft Excel. To estimate circadian rhythm parameters, we used the Microsoft Excel Solver to estimate the optimal parameters for mesor, amplitude, period and phase, to achieve a maximal Pearson’s correlation coefficient to the idealized curve. This was converted to a significance value by applying the Student’s t -distribution equation. Whole-lung flow cytometric analysis Mice were placed in constant dark conditions at CT12 on the day before each experiment. At 4- to 6-h intervals, isofluorane-anaesthetized mice were perfused with 5 ml cold PBS, and their lungs and spleen were manually dissected, minced and dissociated in digestion solution (RPMI 1640, 1.25 mg ml −1 Liberase TM, 30 μg ml −1 DNase I (Roche)). Digested lung was strained through a 100-μm filter (Fischer) and cell yield was determined using a TC10 counter (BioRad). Live cells (250,000–500,000 per well) were then dispensed into 96-well plates and stained live with fluorescently conjugated antibodies (see Supplementary Table 3 for a list of antibodies). The cells were fixed with 1% paraformaldehyde and analysed using a BD Canto II flow cytometer (50,000 events per sample). Data analysis was conducted using FlowJo 7.6.5 software (Tree Star). Please see Supplementary Fig. 10 for representative gates. For each independent experiment, cell counts were normalized to the mesor to control for differences in flow cytometer calibration between sessions. For statistical analysis and rhythm parameter analysis, we used one-way ANOVA and the Microsoft Excel solver as above. Lung immunohistochemistry Non-perfused right lower lobe (RLL) lung fragments were fixed by immersion in 2% paraformaldehyde, paraffin embedded and stained at once using a Leica Bond automated system and antibodies to CD45, B220, MPO or CD31/PE-CAM per standard protocol (see Supplementary Table 4 for a list of antibodies and processing conditions). Slides were then digitally scanned at × 40 using an Aperio ScanScope XT [57] . The entire region of lung from two to three animals per time point was then quantified for positive antibody staining using Aperio ImageScope software and the algorithm ‘Positive Pixel Count v9’. Assuming cell volumes are relatively constant, the fraction of categorically positive pixels will correlate to cell number when averaged over large areas of tissue (to adjust for differences in the plane of sectioning between samples). We used three different thresholds for pixel positivity (provided by the commercial algorithm) to ensure pixel intensity did not affect our relative quantification of cell number. Data were analysed via one-way ANOVA and COSOPT in Microsoft Excel. Metabolite measurements Flash-frozen lung samples ( n =3 per time point) obtained from the first 48 h of observation in Microarray Experiment 2 were analysed by Metabolon using their well-established platform and methods [22] . Relative metabolite abundances were scaled to the median ion count obtained for each metabolite and values that were less than assay were imputed as the lowest measured value per metabolite (please refer to Supplementary Data 19 for scaled and imputed metabolomics data). Of the 395 metabolites that were detected, we excluded 55 because of an excess number of sub-threshold right lower lobe (RLL) assay measurements (by our criteria more than two imputed values in >3 time points), leaving 340 species for analysis. For each metabolite, the data were pre-screened by ANOVA, both as a full time series and with day 1 and 2 of observations pooled (threshold P -value <0.05 in either binning strategy and the best P -value obtained for a given metabolite was the one used). To ensure that data imputation did not affect our conclusions, we excluded metabolites whose significance on ANOVA became subpar when the imputed values were removed. Metabolites passing the ANOVA pre-screening were then analysed by COSOPT and autocorrelation. Because of an excess of imputed values for NAD + and NADP + in the Metabolon-generated data set, we measured these metabolites via commercial enzymatic assay kits (Abcam) according to the manufacturer’s instructions. Antibodies for western blot analysis against AMPKα1/2, phospho-AMPKα1/2 (Thr 172), rS6 and phospho-rS6 (Ser 235/236) were obtained from Cell Signaling Technologies. Methodological limitations It is worth noting some limitations to our approach. The focus of this study was circadian–range rhythms, and as such we sampled lungs at 4-h intervals, consistent with prior studies that examined other murine organs. However, mammalian organs also exhibit ultradian rhythms (period lengths of 12 h or less), which require more frequent sampling for reliable detection [58] . As a result, the prevalence of ultradian expression patterns is probably under-represented in our analysis. The rhythm detection techniques used in this study (CYCLE, COSOPT and Autocorrelation) are based on the goodness-of-fit to single-harmonic cosine curves or based on day-to-day symmetry in the mean expression over time. However, other approaches to rhythm detection exist that may be more sensitive for detecting oscillatory patterns that have irregular contours or have small amplitudes [14] , [58] , [59] . Although the biologic validity of the findings we describe do not depend on any single rhythm detection technique, other analytical approaches might expand the yield from future analyses. In this study we used a single dose of endotoxin administered at a fixed time of day. However, endotoxin exhibits temporal variation in potency in mice and in isolated macrophages [40] , [60] . The disruptions in clock-pathway gene expression that we observed were qualitatively similar to those seen in studies that used different endotoxin doses, administration times, serotypes and model organisms [7] , [8] . Therefore, although we cannot rule out that our results might have been affected by the time of endotoxin administration or dose, our overall conclusions about the effects of severe endotoxemia on circadian regulation in the lung are likely to be broadly applicable. Finally, endotoxin represents one method of inducing systemic inflammation among many and, therefore, we cannot state with certainty that all aspects of our conclusions will be precisely replicated in other models or in heterogeneous groups of patients. We chose endotoxin because this stimulus forms the basis for the current perception that molecular timekeeping is suppressed during systemic inflammation, and because there is documentation that endotoxin produces analogous disruptions to clock gene expression in rodents and in humans. Therefore, although our data have direct relevance to current theories, ultimately genome-wide studies in other disease models and patients will be needed to define how far our conclusions can be generalized. How to cite this article: Haspel, J. A. et al . Circadian rhythm reprogramming during lung inflammation. Nat. Commun. 5:4753 doi: 10.1038/ncomms5753 (2014). Accession codes: Microarray expression data described in this paper has been deposited in the NCBI Gene Expression Omnibus (GEO) under accession code GSE59444 .